Porous hypercrosslinked polymer-TiO2-graphene composite photocatalysts for visible-light-driven CO2conversion Significant efforts have been devoted to develop efficient visible-light-driven photocatalysts for the conversion of CO 2 to chemical fuels. The photocatalytic efficiency for this transformation largely depends on CO 2 adsorption and diffusion. However, the CO 2 adsorption on the surface of photocatalysts is generally low due to their low specific surface area and the lack of matched pores. Here we report a well-defined porous hypercrosslinked polymer-TiO 2 -graphene composite structure with relatively high surface area i.e., 988 m 2 g −1 and CO 2 uptake capacity i.e., 12.87 wt%. This composite shows high photocatalytic performance especially for CH 4 production, i.e., 27.62 μmol g −1 h −1 , under mild reaction conditions without the use of sacrificial reagents or precious metal co-catalysts. The enhanced CO 2 reactivity can be ascribed to their improved CO 2 adsorption and diffusion, visible-light absorption, and photo-generated charge separation efficiency. This strategy provides new insights into the combination of microporous organic polymers with photocatalysts for solar-to-fuel conversion. The rapid consumption of carbon-rich fossil fuels has accelerated global energy shortage and significantly increased the CO 2 emissions causing serious environmental issues including greenhouse effect responsible for global warming. Among various strategies for CO 2 conversion, the photoreduction of CO 2 into chemical fuels has attracted increasing attention recently because it utilizes the abundant and sustainable solar energy to mimic the natural photosynthesis [1] , [2] . So far, two approaches, i.e., homogeneous system and heterogeneous system, have been developed for the photoreduction of CO 2 . In homogeneous systems, the molecular metal complexes have shown high photocatalytic reactivity towards CO 2 reduction [3] , [4] , [5] . In contrast, the conversion efficiency in heterogeneous systems is relatively low, and the exploration of high performance heterogeneous photocatalysts is highly desired keeping in view their higher stability and recyclability [6] , [7] . In heterogeneous photocatalytic systems, the electrons are generated by light absorption and then transferred to the catalytically active sites to react with the adsorbed CO 2 molecules, so the conversion efficiency essentially relies on the light absorption ability, generation and separation of the photogenerated charge carriers, and CO 2 adsorption and diffusion [7] , [8] . Tremendous efforts have been made to optimize the structure and composition of semiconductor photocatalysts to improve their visible-visible light absorption and charge separation efficiency, e.g., constructing heterojunctions, creating surface defects, introducing metal co-catalysts, and engineering exposed crystal facets etc [9] , [10] , [11] , [12] , [13] , [14] . The CO 2 adsorption ability is particularly crucial to photocatalytic heterogeneous systems for CO 2 conversion, which readily occurs at the active sites of photocatalysts developing intimate contact with CO 2 molecules [1] , [7] , [15] . Unfortunately, the CO 2 adsorption on the surface of semiconductor photocatalysts is extremely low due to their low specific surface area and the lack of matched pores [7] , [16] . To overcome this limitation, the researchers have modified the photocatalytic reaction systems by elevating pressure, adding sacrificial reagents, or introducing CO 2 -philic solvents [13] , [17] , [18] . In contrast, it is relatively difficult to achieve efficient photocatalytic reduction of CO 2 under mild gas–solid reaction conditions without the use of sacrificial reagent or precious metal co-catalyst, and can be further enhanced by the rational design of the microporous structure to facilitate the CO 2 uptake and conversion. Given this challenge, incorporating a CO 2 capture material into the photocatalytic system has great potential to provide an opportunity for improving CO 2 conversion efficiency. For example, the integration of metal-organic frameworks (MOFs) with photocatalysts has been demonstrated to offer better adsorptive sites for gas uptake because of their larger surface area and microporosity [19] , [20] , [21] . 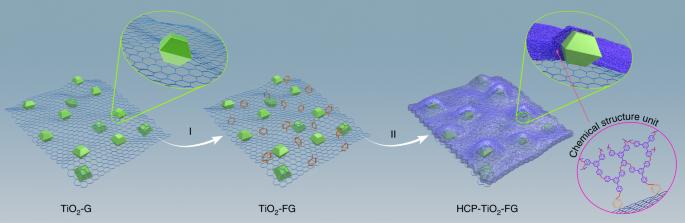Fig. 1 Construction of a well-defined porous HCP-TiO2-FG composite structure. I The functionalization of TiO2-G by diazonium salt formation. II The knitting of TiO2-FG withsyn-PhPh3by solvent knitting method. The magnified model in the top right corner is the cross profile of HCP-TiO2-FG composite Although the CO 2 conversion efficiency has been greatly improved by MOFs incorporation (Supplementary Table 1 ), the photocatalytic performance is still not sufficient for the practical applications, especially because the methane generation is quite limited [22] . It has been established that the prerequisites to CO 2 transformation involve two steps i.e., CO 2 capture and diffusion to the catalytic sites [7] , [15] . The porous capture materials possess abundant adsorptive sites but they are less catalytically active for CO 2 reduction than semiconductors or precious metals [23] . Thus the photoreduction efficiency largely depends on the CO 2 diffusion from the capture materials to the photocatalysts [19] . Therefore, in order to achieve higher CO 2 conversion, an efficient photocatalyst requires high CO 2 uptake as well as short diffusion length. As a proof of concept, we develop a porous composite structure by in situ knitting hypercrosslinked polymers (HCPs) on TiO 2 -functionalized graphene (TiO 2 -FG). The HCPs materials as pure organic microporous materials show large surface area, high CO 2 uptake, and excellent physicochemical stability [24] . It is worth mentioning that this is the example involving the combination of microporous organic polymers with photocatalysts for CO 2 conversion among the numerous reported photocatalysts. The synthetic strategy of such well-defined porous composite structure is depicted in Fig. 1 . The TiO 2 -G composite is initially obtained by the reduction of graphene oxide (GO) followed by in situ growth of the anatase TiO 2 crystals with reactive {001} facets on its surface by a solvothermal process [25] , [26] . The graphene skeleton of TiO 2 -G composite is functionalized to form TiO 2 -FG and provide an open phenyl group for covalent linking (step I). Finally, the ultrathin polymer layers are hypercrosslinked on TiO 2 -FG by the knitting of syn -PhPh 3 and the open phenyl groups on graphene (step II), resulting in the formation of the porous hypercrosslinked polymer-TiO 2 -graphene (HCP-TiO 2 -FG) composite [27] , [28] . Due to the enhanced CO 2 adsorption ability of HCPs and the short diffusion length around the TiO 2 photocatalysts, such well-defined HCP-TiO 2 -FG structure is envisioned to enhance the reactivity of CO 2 molecules to facilitate the production of CH 4 . Fig. 1 Construction of a well-defined porous HCP-TiO 2 -FG composite structure. I The functionalization of TiO 2 -G by diazonium salt formation. II The knitting of TiO 2 -FG with syn -PhPh 3 by solvent knitting method. The magnified model in the top right corner is the cross profile of HCP-TiO 2 -FG composite Full size image Characterization of the resulting materials The morphology and microstructure of the as-prepared materials were investigated by transmission electron microscopy (TEM), field-emission scanning electron microscopy (FE-SEM), and atomic force microscopy (AFM). FE-SEM characterization of pure HCPs from our previous knitting method showed a layered bulk structure [27] , [28] , whereas the HCP-TiO 2 -FG exhibited a 3D morphology with flake-like graphene sheets, which is similar to the reported porous graphene-based materials [29] , [30] . The absence of naked TiO 2 crystals on the graphene surface indicated their complete coating by the HCPs layers in HCP-TiO 2 -FG (Supplementary Figure 1a–d ). 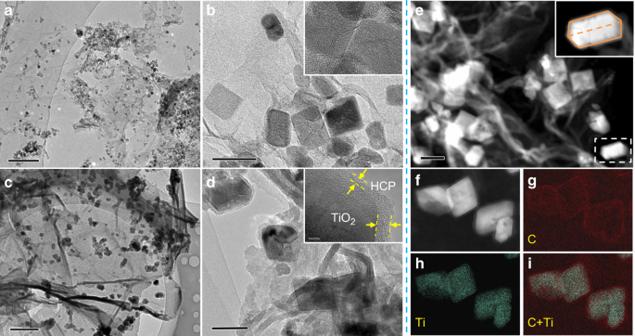Fig. 2 Morphology and elemental mapping of various photocatalysts. TEM images ofa,bTiO2-G andc, dHCP-TiO2-FG at different magnification. The insets inbanddare the corresponding HR-TEM images.eSTEM image of HCP-TiO2-FG.f–iHigh-angle annular dark field (HAADF) mapping images of HCP-TiO2-FG. The scale bar are 200 nm ina, 50 nm inb, 0.5 μm inc, 100 nm ind, 100 nm ine, and 5 nm in insets inbandd The TEM characterization further showed that the smooth graphene nanosheets (Supplementary Figure 2 ) were uniformly decorated with TiO 2 crystals to confirm the formation of TiO 2 -G composite nanostructure (Fig. 2a,b ). After in situ knitting, a distinct composite structure was formed of HCP-TiO 2 -FG in which the graphene surface and TiO 2 crystals were covered by the HCPs layers. No freestanding HCPs blocks were observed in SEM, TEM, and scanning transmission electron microscopy (STEM) images (Fig. 2c–e and Supplementary Figure 1d ). High-resolution TEM (HR-TEM) characterization showed that the TiO 2 crystals were fully wrapped by an ultrathin HCPs layer with a thickness of 3–8 nm (Fig. 2d ). The typical AFM observation and thickness analysis revealed a uniform thickness of HCP-TiO 2 -FG as 10 ± 0.5 nm, whereas the thickness of TiO 2 -FG was only 4 ± 0.5 nm suggesting the formation of composite structure (Supplementary Figures 3 – 4 ). The percentage of the exposed {001} facets in the TiO 2 crystal was calculated to be ~30% using a geometric calculation (Supplementary Figure 5 ). The elemental mapping images in Fig. 2f–i clearly display the thin HCP shells wrapping the surface of TiO 2 crystals. By rotating the angle of the sample, multiple images were collected to create a three-dimensional TEM (3D-TEM) movie (Supplementary Figure 6 and Supplementary Movie 1 ) to further elucidate the HCP-TiO 2 -FG composite structure with distinct interface between TiO 2 and HCP-FG. Based on the above analysis, it can be deduced that the TiO 2 crystals were supported on the graphene sheets and then encapsulated by the ultrathin HCPs layers after knitting syn -PhPh 3 with functionalized graphene, as shown in Fig. 1 . Fig. 2 Morphology and elemental mapping of various photocatalysts. TEM images of a , b TiO 2 -G and c, d HCP-TiO 2 -FG at different magnification. The insets in b and d are the corresponding HR-TEM images. e STEM image of HCP-TiO 2 -FG. f–i High-angle annular dark field (HAADF) mapping images of HCP-TiO 2 -FG. The scale bar are 200 nm in a , 50 nm in b , 0.5 μm in c , 100 nm in d , 100 nm in e , and 5 nm in insets in b and d Full size image The X-ray diffraction (XRD) pattern showed that all the samples consisted of pure anatase TiO 2 crystals. The introduction of HCPs layers did not alter the crystal phase of TiO 2 but caused an obvious increase in the particle size (Fig. 3a ), which followed the Ostwald ripening mechanism during long-time refluxing in the functionalization and knitting processes. The composition and surface chemical structure were investigated by X-ray photoelectron spectroscopy (XPS) measurements. Unlike TiO 2 -G, the peak intensities of Ti and O signals for TiO 2 -FG and HCP-TiO 2 -FG were gradually weakened due to the decrease of TiO 2 content (Supplementary Figure 7a ). As shown in high-resolution C 1s spectra, the ratio of sp 2 C and sp 3 C signals demonstrated an increasing trend after functionalization and knitting, which was attributed to the introduction of more sp 2 C compared with the formation of sp 3 C (Fig. 3b and Supplementary Figure 7b,c ) [30] . Interestingly, the location of Ti 2p displayed an obvious shift of ~0.2 eV towards higher energy after HCPs layers formation (Supplementary Figure 7d ). This shift verified the electronic interaction of HCPs layers with TiO 2 , which was favorable for the electron transfer at the heterojunction interface. Fourier transform infrared (FT-IR) spectroscopy was carried out to investigate the chemical structure of the resulting materials. Compared with the FT-IR spectrum of TiO 2 -FG, strong C–H stretching vibrations of methylene near 2920 cm −1 and aromatic ring skeleton vibration peaks near 1485 cm −1 are clearly visible for HCP-TiO 2 -FG (Supplementary Figure 8 ) [27] , [28] . The slight shift of the Ti-O-Ti stretching vibration further verified the interfacial interactions of TiO 2 with HCPs layers in the composite materials. Fig. 3 Chemical structure, porosity, and CO 2 uptake of various photocatalysts. a XRD image of TiO 2 , TiO 2 -G, and HCP-TiO 2 -FG. b C 1s profiles of HCP-TiO 2 -FG. c 13 C cross-polarization/magic-angle spinning (CP/MAS) NMR spectra of HCP-TiO 2 -FG. d Nitrogen adsorption and desorption isotherms at 77.3 K of samples. e Volumetric CO 2 adsorption isotherms and desorption isotherms up to 1.00 bar at 273.15 K of samples. f Volumetric CO 2 adsorption isotherms and desorption isotherms up to 1.00 bar at 298.15 K of samples Full size image The 13 C cross-polarization/magic-angle spinning nuclear magnetic resonance (CP/MAS NMR) was employed to further confirm the proposed functionalization and knitting processes at the molecular level. The introduction of phenyl groups in TiO 2 -FG resulted in the appearance of a shoulder peak arising at 136.7 ppm in the aromatic carbon region due to the functionalization of TiO 2 -G, and the resonance at 127.2 ppm are assigned to the sp 2 carbons of the graphene based on reported data (Supplementary Figure 9 ) [30] . The enhanced intensity of resonance peaks near 136.7 ppm can be ascribed to the introduction of abundant sp 2 carbon by knitting syn -PhPh 3 with TiO 2 -FG for HCP-TiO 2 -FG. Meanwhile, the methylene linkers formed by knitting processes resulted in the appearance of a new peak near 32.9 ppm (Fig. 3c ) [27] , [28] . The TiO 2 content and thermostability of as-prepared materials were investigated by thermogravimetric analysis (TGA). As expected, the percent weight loss of TiO 2 significantly decreased from the initial 67% for TiO 2 -G to 31% for HCP-TiO 2 -FG suggesting the incorporation of HCPs layers into the composite (Supplementary Figure 10 ). The results are in good agreement with the accurate measurement by inductively coupled plasma-mass spectrometry (ICP-MS) analysis. More importantly, the HCP-TiO 2 -FG composite structure exhibited the excellent thermal stability comparable to TiO 2 -G with resistance to degradation up to 400 °C, presumably due to the formation of HCPs layers on rigid graphene skeletons. Porosity and CO 2 uptake of the resulting materials After confirming the morphology and chemical structure of the as-prepared materials, we further investigated their porosity parameters as shown in Fig. 3d and Supplementary Table 2 . The TiO 2 and TiO 2 -FG showed type IV isotherms with a minute amount of adsorbed nitrogen and obvious hysteresis loops at medium pressure region, indicating low surface area and the existence of mesopores [31] , [32] . The isotherms of HCP-TiO 2 -FG exhibited a type I character with a steep nitrogen gas uptake at low relative pressure ( P/P 0 < 0.001) thus reflecting abundant microporous structure. The existence of an obvious hysteresis and a slight rise at medium and high pressure region revealed the presence of mesopores and macropores, respectively [33] . 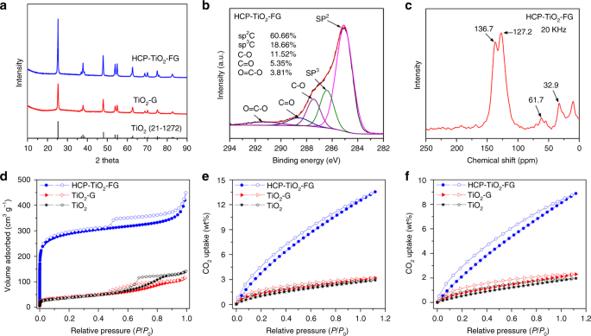Fig. 3 Chemical structure, porosity, and CO2uptake of various photocatalysts.aXRD image of TiO2, TiO2-G, and HCP-TiO2-FG.bC1sprofiles of HCP-TiO2-FG.c13C cross-polarization/magic-angle spinning (CP/MAS) NMR spectra of HCP-TiO2-FG.dNitrogen adsorption and desorption isotherms at 77.3 K of samples.eVolumetric CO2adsorption isotherms and desorption isotherms up to 1.00 bar at 273.15 K of samples.fVolumetric CO2adsorption isotherms and desorption isotherms up to 1.00 bar at 298.15 K of samples More importantly, the introduction of HCPs layers dramatically enlarged the specific surface area of TiO 2 -G to 988 m 2 g −1 , together with an increase in micropore volume from 0.009 to 0.306 cm 3 g −1 , which is, in fact, much higher than the reported semiconductor-graphene composites or most of the porous photocatalysts (Supplementary Table 3 ). Moreover, the dominant pore diameter of HCP-TiO 2 -FG was centred at about 0.5 and 1.1 nm, along with continuous mesoporous and macroporous structure (Supplementary Figure 11 ). The high specific surface area and abundant ultra-microporous nature of the HCP-TiO 2 -FG composite inspired us to investigate its gas uptake capacity. It is well established that the CO 2 uptake by porous polymer materials mainly results from its physical adsorption [34] , [35] . Such adsorption mode displays the pressure and temperature-dependent features with excellent recyclability for the repeated CO 2 adsorption and desorption (Supplementary Figure 12 ). Interestingly, the CO 2 uptake of the HCP-TiO 2 -FG reached as high as 12.87 wt% at 1.00 bar and 273.15 K, which is more than four-fold higher than those of TiO 2 and TiO 2 -G. These results were finally compared with some porous photocatalysts reported under similar conditions (Fig. 3e,f and Supplementary Table 3 ). It was found that the CO 2 uptake of HCP-TiO 2 -FG was higher than that of HCP-FG (Supplementary Table 2 ), implying that the TiO 2 intercalation somewhat restricted the aggregation of HCPs layers on graphene nanosheets. To further understand the effect of such well-defined HCP-TiO 2 -FG composite structure on improving surface area and CO 2 uptake, another type of composite, TiO 2 /HCP-FG, was prepared as a control by changing the order of introducing HCP and TiO 2 . The HCP layers were hypercrosslinked on the functionalized graphene to form HCP-FG at first, and then TiO 2 crystals were grown on the HCP-FG surface during the solvothermal process. Owing to the high surface area and porous property of HCP-FG support, the TiO 2 particles of TiO 2 /HCP-FG possessed much smaller size than that of TiO 2 -G or HCP-TiO 2 -FG (Supplementary Figure 13 ). However, the hypercrosslinking reaction caused the graphene surface to be almost entirely covered by HCP layers, so that most of TiO 2 crystals were assembled on the HCP surface rather than be encapsulated by HCPs layers like those in HCP-TiO 2 -FG composite. The results implied the interaction of TiO 2 with graphene serving as bridge to the formation of well-defined HCP-TiO 2 -FG composite structure. The TiO 2 /HCP-FG composite showed a high surface area of 178 m 2 g −1 and CO 2 uptake of 3.31 wt% relative to TiO 2 and TiO 2 -G (Supplementary Figure 14 ), but much lower than that of HCP-TiO 2 -FG. According to the previous such reports, the incorporation of semiconductor photocatalysts generally decrease the surface area and CO 2 uptake of the capture materials, mainly resulting from the semiconductors with low surface area occupying the porous surface [19] , [23] , [36] , [37] . Hence the superiority of HCP-TiO 2 -FG in CO 2 adsorption could be ascribed to the well-defined porous composite structure with TiO 2 encapsulated inside the HCP-FG network instead of being assembled on the surface. Photoreduction CO 2 activity of the resulting materials Given ideal pore distribution and excellent CO 2 capture capacity of HCP-TiO 2 -FG, we set out to evaluate the photocatalytic efficiency towards CO 2 conversion in a gas–solid reaction system. The photoreduction of CO 2 proceeded under mild conditions without any photosensitizer or organic sacrificial reagent. 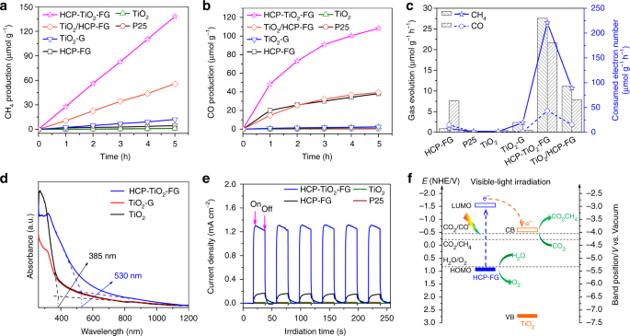Fig. 4 The photocatalytic performance of CO2reduction, optical and photoelectrical properties, and mechanism of charge transfer pathway. Time-dependent production ofaCH4andbCO in photocatalytic CO2reduction with different catalysts under visible-light (λ≥ 420 nm). The photocatalytic reactions were carried out in a batch system under standard atmospheric pressure. The partial pressure of CO2and H2O were constant with the water contents below the scaffold loading photocatalyst. Under visible-light irradiation, the temperature of the water was measured to be about 50 °C.cAverage efficiency of photocatalytic CO2conversion with different catalysts during 5 h of visible-light (λ≥ 420 nm) irradiation.dUV-Vis absorption spectra of TiO2, TiO2-G, and HCP-TiO2-FG catalysts.eAmperometricI−tcurves of samples under visible-light (λ≥ 420 nm) irradiation.fProposed mechanism of charge separation and transfer within the HCP-TiO2-FG composite photocatalyst under visible-light (λ≥ 420 nm) irradiation Figure 4a,b and Table 1 show the yield of the CO 2 conversion products during 5 h of photocatalytic reaction under visible-light (wavelength λ ≥ 420 nm) irradiation. The CO and CH 4 gases were generated as main products via the two-electron and eight-electron reduction processes, respectively. The porous HCP-TiO 2 -FG catalyst presented high average conversion efficiency with a rate of total consumed electron number ( R e ) as 264 μmol g −1 h −1 , a CH 4 evolution rate of 27.62 μmol g −1 h −1 , and a CO evolution rate of 21.63 μmol g −1 h −1 . Figure 4c shows the dominant electron consumption selectivity for CH 4 production as high as 83.7%. More importantly, no H 2 evolution was detected during the photocatalytic reaction suggesting that the HCP-TiO 2 -FG material possessed the high selectivity for photoreduction of CO 2 and effectively hindered the side reaction of H 2 O reduction. To the best of our knowledge, these CO 2 photoconversion results are the best among those of the recently reported heterogeneous photocatalysts under similar gas–solid reaction conditions (with no sacrificial reagent), especially much higher than those of photocatalysts without precious metal co-catalysts (Supplementary Table 1 ) [11] , [17] , [23] , [38] , [39] , [40] . Fig. 4 The photocatalytic performance of CO 2 reduction, optical and photoelectrical properties, and mechanism of charge transfer pathway. Time-dependent production of a CH 4 and b CO in photocatalytic CO 2 reduction with different catalysts under visible-light ( λ ≥ 420 nm). The photocatalytic reactions were carried out in a batch system under standard atmospheric pressure. The partial pressure of CO 2 and H 2 O were constant with the water contents below the scaffold loading photocatalyst. Under visible-light irradiation, the temperature of the water was measured to be about 50 °C. c Average efficiency of photocatalytic CO 2 conversion with different catalysts during 5 h of visible-light ( λ ≥ 420 nm) irradiation. d UV-Vis absorption spectra of TiO 2 , TiO 2 -G, and HCP-TiO 2 -FG catalysts. e Amperometric I − t curves of samples under visible-light ( λ ≥ 420 nm) irradiation. f Proposed mechanism of charge separation and transfer within the HCP-TiO 2 -FG composite photocatalyst under visible-light ( λ ≥ 420 nm) irradiation Full size image Table 1 Summary of the photocatalytic CO 2 conversion efficiency during 5 h of constant irradiation Full size table The well-defined HCP-TiO 2 -FG composite photocatalyst with abundant microporosity demonstrated excellent performance for CO 2 reduction but its underlying mechanism still needs to be investigated. The CO 2 conversion products were rarely detected (<1 μmol g −1 h −1 ) over commercial TiO 2 (P25), and pure TiO 2 with reactive {001} facets due to their limited light-responsive ability in the visible region (Fig. 4d ). Coupling of TiO 2 with graphene to produce TiO 2 -G obviously increased the CH 4 production (2.42 μmol g −1 h −1 ) by improving visible-light absorption and electron transport property [18] , [41] . The adsorptive and catalytic sites can be clarified through the comparison in porous property and photocatalytic performance. Obviously, the introduction of porous HCPs layers enriched the adsorptive sites to achieve the high CO 2 uptake and improved the visible light absorption. Thus the formation of well-defined HCP-TiO 2 -FG composite structure resulted in much higher photocatalytic CO 2 reduction rate. The HCP-FG material also exhibited broad visible-light absorption, high surface area, and notable CO 2 uptake (Supplementary Table 2 ). However, its photocatalytic performance was far less than that of HCP-TiO 2 -FG, especially in the eight-electron reduction to CH 4 (Fig. 4a and Table 1 ). It is well known that the polymer materials usually possess the excitons with high binding energy, which usually recombine at the excited states [42] . That is, the adsorptive sites on the porous capture material are generally catalytically inactive for CO 2 reduction [23] . To further elucidate the superiority of porous HCP-TiO 2 -FG composite, the CO 2 conversion efficiency over TiO 2 /HCP-FG composite was evaluated. It was found that the photocatalytic activity of TiO 2 /HCP-FG was much lower than that of HCP-TiO 2 -FG. It may be due to the blockage of the porous structure of HCP-FG with TiO 2 crystals thereby decreasing the surface area and CO 2 uptake and subsequently leading to the reduced CO 2 reduction rate. Although TiO 2 deposition blocked most of the adsorptive sites of HCP-FG and resulted in a dramatic decrease to less than one-third of CO 2 uptake, the CH 4 production over TiO 2 /HCP-FG was, however, 7.4 times more than that over pristine HCP-FG. The comparison among HCP-FG, HCP-TiO 2 -FG, and TiO 2 /HCP-FG shows that the catalytic sites on TiO 2 are much more active for CO 2 reduction than those on HCP-FG. The model of CO 2 diffusion and conversion is presented in Supplementary Figure 15 . Based on the above analysis, it can be deduced that the in situ knitting strategy for HCP-TiO 2 -FG can effectively produce porous structure without significant pore blockage of the porous polymers. More importantly, the HCPs obtained by this strategy are comprised of ultrathin layers with a thickness of 3–8 nm wrapping around TiO 2 crystals (Fig. 2d–f ), which facilitates the diffusion of CO 2 molecules from the adsorptive sites on HCPs layers to the catalytic sites on TiO 2 photocatalysts. The effect of the thickness of HCP layers on the CO 2 conversion efficiency was studied by adjusting the amount of syn -PhPh 3 . By increasing the amount of syn -PhPh 3 , the mass ratio of TiO 2 was slightly decreased from 31 to 29% (Supplementary Figure 16 ), however, the size of TiO 2 particles was decreased accompanied by the thickening of the HCP layers (Supplementary Figure 17 ), which suggests that the HCP outer layers effectively suppress the growth of TiO 2 crystals. The distinct thickening of the outer layers was further verified from the characteristic morphology revealed in Fig. 1 , showing HCP layers being hypercrosslinked on FG surface and encapsulating TiO 2 crystals. The surface area and CO 2 uptake capacity increased with the amount of syn -PhPh 3 (Supplementary Figure 18a and Supplementary Table 4 ), on the other hand, the diffusion length of CO 2 molecules also increased due to the thickening of the outer layer. As the CO 2 conversion efficiency increased initially and then decreased at higher amount (Supplementary Figure 18b ), there may be an appropriate thickness of HCP layers that balance the CO 2 adsorption and diffusion. As a result of the relatively high photocatalytic performance of porous HCP-TiO 2 -FG, the O 2 evolution can be measured to provide the evidence of the oxidation cycle offering a better insight of the mechanism that is seldom discussed in the literature [43] . The O 2 evolution rate over HCP-TiO 2 -FG under visible-light irradiation was determined to be 1.6 μmol h −1 , while the O 2 evolution over other photocatalysts was too low to be detectable (Supplementary Figure 19 ). The electrons from the water oxidation are slightly higher than the total consumed electrons for the reduced products including CH 4 and CO. To verify the evolution of CO and CH 4 from CO 2 conversion over HCP-TiO 2 -FG photocatalyst, we conducted three controlled experiments: (1) irradiation of catalyst under inert N 2 condition; (2) the use of isotopically labeled 13 CO 2 and H 2 18 O as the reactants; (3) irradiation of catalyst in the presence of CO 2 gas without H 2 O vapors. Under inert N 2 condition, no CH 4 was detected and the CO yield was only 7% compared to that under CO 2 atmosphere (Supplementary Figure 20 ). The trace CO product might be generated by the decomposition of the residual oxygen-containing functional groups of graphene, which was evidenced by XPS analysis (Supplementary Figure 7a ). In an isotopically labeled experiment, the 13 CH 4 and 13 CO signals at m/z = 17 and m/z = 29 appeared after the photocatalytic reaction. The results confirmed that the CO and CH 4 products are indeed originating from the photocatalytic reduction of CO 2 gas (Supplementary Figure 21 ). The isotopically labeled H 2 18 O vapors led to the formation of 18 O 2 (Supplementary Figure 22 ), suggesting that the evolved O 2 gas was derived from the photocatalytic water oxidation. In the absence of H 2 O vapors, the CH 4 evolution was rapidly declined to ~9% of the original rate, while ~1.8 times increase was observed in CO evolution, revealing that the H 2 O vapors act as the proton donors for the conversion of CO 2 to CH 4 [44] . Although the porous HCP-TiO 2 -FG also exhibits a high adsorption capacity towards water vapors, about 30 wt% at 90% humidity (Supplementary Figure 23 ), the existence of water vapors brings a slight increase in CO 2 uptake (Supplementary Figure 24 ), presumably due to their affinity with the water molecules. The CH 4 evolution is relatively difficult since the reactivity of the adsorbed CO 2 molecules should be high enough to accept eight electrons and eight protons to break the C–O bonds and form the C–H bonds [45] . Normally, the adsorbed CO 2 molecules are more readily converted to CO than CH 4 on the surface of semiconductor photocatalysts [18] , [19] , [36] . Precious metal co-catalysts are generally introduced to improve the reactivity of CO 2 molecules to obtain more CH 4 production, e.g., 19.6 μmol g −1 h −1 over Pd 7 Cu 1 -loaded TiO 2 and 20.6 μmol g −1 h −1 over TiO 2 -PdH 0.43 under UV-light [40] , [46] . However, the CH 4 evolution over the HCP-TiO 2 -FG (this study) under UV-light can achieve a high rate of 51.23 μmol g −1 h −1 (Supplementary Figure 25 ). To the best of our knowledge, the CH 4 evolution rate over the HCP-TiO 2 -FG under UV- or visible-light irradiation is impressively higher than the reported values including that over precious metal-modified TiO 2 photocatalysts (Supplementary Table 1 ), under similar gas–solid reaction conditions (with no sacrificial agent). The charge separation efficiency was investigated by recording the transient amperometric I - t curves under visible-light irradiation. As shown in Fig. 4e , the photocurrent of the resulting materials displayed high repeatability during light on-off cycling, and the results were consistent with the photocatalytic evaluations, i.e., negligible signal in pure TiO 2 system, weak photocurrent response in HCP-FG, and notably enhanced current intensity in HCP-TiO 2 -FG composite. The photoluminescence (PL) and electrochemical impedance spectra (EIS) were employed to provide further evidence as shown in Supplementary Figures 26 – 27 . The significant PL quenching suggests that the recombination of the photogenerated e − /h + pairs was effectively suppressed by graphene. The smaller semicircle arc at high frequencies in the EIS indicates the decreased electron-transfer resistance ( R et ) across the electrode/electrolyte. The lower R et of TiO 2 -FG than that of TiO 2 indicates that FG modification favors the electronic conductivity due to its high electron mobility. Moreover, the covalent linking with graphene effectively improves the electronic conductivity of the HCPs and thus facilitates the electron transfer in the composite. The less efficient CH 4 production over HCP-TiO 2 photocatalyst can also reflect the influence of graphene on improving the charge separation efficiency (Supplementary Figure 28 ). As a result, the porous HCP-TiO 2 -FG composite possesses the improved efficiency in separating the photogenerated charge carriers. The pathway of charge carriers transfer and separation generally depends on the band gap of photocatalysts. The HCP-FG showed that its highest occupied molecular orbital (HOMO) and lowest unoccupied molecular orbital (LUMO) energy levels were located at −5.34 eV and −3.00 eV (vs. vacuum level) as calculated by optical absorption (Fig. 4d ) and cyclic voltammetry (CV) measurement (Supplementary Figure 29 ), which are more negative than the valence band (VB) and conduction band (CB) levels of TiO 2 , respectively. To further confirm, ultraviolet photoelectron spectroscopy (UPS) technique was employed to measure the HOMO location, −5.44 eV vs vacuum level (Supplementary Figure 30 ), which was found to be very close to that of CV measurement. Based on the position of HOMO and LUMO energy levels, a tentative mechanism for the overall CO 2 conversion process over the HCP-TiO 2 -FG photocatalyst is proposed and is shown in Fig. 4f . Under visible-light irradiation, HCP-FG functions both as CO 2 adsorbent and photosensitizer, which directly absorbs the photons to induce the HOMO to LUMO transition. The photogenerated electron-hole pairs of the excited HCP-FG can migrate and separated at the interface with TiO 2 via their interfacial interaction, as shown in Supplementary Figure 31 . Thus the CO 2 reduction is inclined to occurr at the catalytic sites on TiO 2 rather than that on HCP-FG, which is in consistent with the above discussions on the porous property and photocatalytic performance. The electron transfer not only largely inhibited the recombination with the excited HCP-FG, but also made the photocatalytic reaction more effective. The excited HCP-FG was recovered to its neutral state by oxidizing the absorbed water molecules to produce oxygen gas. When the light was turned off, the amount of CO and CH 4 remained almost constant, indicating the efficient control over the reverse reactions of CO 2 reduction (oxidizing CO and CH 4 to CO 2 ) over the HCP-TiO 2 -FG photocatalyst under such mild reaction conditions (Supplementary Figure 32 ). It can be concluded that the in situ knitting of porous HCP-TiO 2 -FG are very effective to dramatically enhance visible-light-driven CO 2 conversion efficiency, which could be mainly ascribed to the well-defined composite structure from the following two aspects: (1) high CO 2 uptake ability and short distance between the adsorbent and the catalyst facilitating the CO 2 adsorption and diffusion; (2) broad light absorption of HCPs layers and fast charge mobility of graphene improving the visible-light absorption and charge separation efficiency. In this way, the high selectivity of electron consumption for CH 4 production can also be explained by the enrichment of CO 2 and electron density favoring the multi-electron reduction process. In addition to the enhanced photocatalytic activity, the stability of such photocatalysts is also crucial for composite structure because of the possible leakage of one component from another. It was observed that HCP-TiO 2 -FG retained more than 85% of the original efficiency for both the CH 4 and CO production, implying their stable framework by strong interfacial interaction after five consecutive runs (Supplementary Figure 33 ). Moreover, the fresh and used catalysts displayed no obvious difference in FT-IR spectra and XRD diffraction pattern, which demonstrates the stable chemical skeleton and crystal structure of HCP-TiO 2 -FG throughout the photocatalytic reaction (Supplementary Figures 34 – 35 ). Kinetic analysis The kinetics experiments were carried out to understand the contribution of CO 2 adsorption and diffusion to the enhancement of photocatalytic efficiency. The relationship between the CO 2 adsorption and CH 4 production can be explored by varying the surface coverage of CO 2 on the active sites. The partial pressure of CO 2 is adjusted in CO 2 /N 2 mixture because of a high CO 2 /N 2 selectivity ratio of 25.8 over the HCP-TiO 2 -FG photocatalyst (Supplementary Figure 36 ). Since the kinetic model and reaction mechanism of photocatalytic CO 2 conversion are ambiguous so far, the quantitative relationship between CO 2 coverage and CH 4 evolution rate is still unclear. Interestingly, it is observed that they show a similar trend of increase with CO 2 proportion, e.g., both of them dramatically increased at lower partial pressure and then displayed a slow increase at higher CO 2 concentration (Supplementary Figure 37 ). Generally, the reaction rates that are normalized to the active sites allow the direct comparison of intrinsic reactivity on different catalysts [47] , [48] , [49] . For the catalytic system employing same catalyst, the reaction rate appears to be independent of the loading amount of catalyst after normalization to the same amount [50] , [51] . In this regard, the porous HCP-TiO 2 -FG photocatalyst possesses equivalent catalytic active sites to TiO 2 /HCP-FG due to the same content of TiO 2 photocatalyst. That is, the more efficient CH 4 production over HCP-TiO 2 -FG should not result from the difference in the number of catalytic sites but mostly come from the higher surface coverage of CO 2 on the active sites. The temperature has a complicated influence on the rate of photocatalytic conversion from the aspects of adsorption and diffusion. By increasing the temperature, the surface coverage of CO 2 molecules on the catalyst surface was decreased due to the exothermic effect of adsorption process (Fig. 3 e–f), while the diffusion rate was increased as a result of the increased thermal motion of CO 2 molecules (Supplementary Figure 38 ). Based on Arrhenius plot, the adsorption activation energy for CO 2 adsorption is calculated to be 5.20 kJ mol −1 (Supplementary Figure 39a ) using a microporous diffusion model [52] , [53] . Since the CH 4 production increases linearly and possesses dominant electron consumption selectivity as 83.7%, we can use the pseudo-zero-order model to estimate the rate constant for the overall reaction, obtaining apparent activation energy of 9.34 kJ mol −1 (Supplementary Figure 39b ). The diffusion process was further studied by varying the stirring speed. As shown in Supplementary Figure 40 , the increase of stirring speed greatly facilitates the photocatalytic conversion of CO 2 to CH 4 product. Combining the diffusion effect with pressure-/temperature-dependent characteristics, we can conclude that the photocatalytic CO 2 reduction over HCP-TiO 2 -FG is not under intrinsic kinetic control of the catalyst, but the efficiency is rather determined by gas adsorption and diffusion. The elucidation of adsorption and diffusion that contributed to the photocatalytic reaction, and is seldom discussed in the literature, provides valuable information for understanding the relationship between the catalytic performance and structure properties. As a result, it clearly demonstrates the superiority of such porous HCP-TiO 2 -FG composite towards the visible-light-driven photocatalytic CO 2 conversion. Further kinetic study is required to probe the kinetics model and reaction mechanism of photocatalytic CO 2 conversion. In summary, the well-defined porous HCP-TiO 2 -FG composite structure was successfully constructed by in situ knitting strategy. The anatase TiO 2 crystals with reactive {001} facets were supported on graphene surface and encapsulated inside the ultrathin HCPs layers with a thickness of 3–8 nm. Benefiting from the high surface area and abundant microporous nature, the introduction of HCPs layers dramatically improved the specific surface area and micropore volume of TiO 2 -G to 988 m 2 g −1 and 0.306 cm 3 g −1 , respectively, leading to the increased CO 2 uptake capacity up to 12.87 wt%. Due to the improved CO 2 adsorption ability and shortened diffusion length, such well-defined HCP-TiO 2 -FG composite photocatalyst is expected to enhance the reactivity of CO 2 molecules, which will facilitate the CO 2 conversion especially for CH 4 production. In addition, the charge separation efficiency and visible-light absorption of TiO 2 photocatalyst could be effectively improved by the graphene with high charge mobility and the HCPs layers with broad light absorption. As a result, the HCP-TiO 2 -FG achieved high CO 2 conversion efficiency with a rate of total consumed electron number ( R e ) as 264 μmol g −1 h −1 , including 83.7% selectivity for CH 4 production and negligible side reaction of H 2 production under visible-light irradiation. To the best of our knowledge, these results are the best among the recent such reports, and especially much better than those of photocatalysts with precious metal co-catalysts under similar gas–solid reaction conditions. We believe that these findings will be very helpful to overcome the constraint of deficient pore structure for semiconductor-based composites and open a new pathway for the design and synthesis of well-defined porous materials with high CO 2 uptake and photocatalytic conversion efficiency. Materials Graphite, isopropyl alcohol, dichloromethane, hydrochloric acid, fluoric acid, ethanol, AlCl 3 (anhydrous), H 2 SO 4 , NaNO 3 , KMnO 4 , and K 2 CO 3 were obtained from National Medicines Corporation Ltd. of China, all of which were of analytical grade and were used as received. 1, 3, 5-triphenylbenzene ( syn -PhPh 3 ), tetrabutyl titanate, isoamyl nitrite, and aniline were purchased from Aladdin chemical reagent Corp (Shanghai, China) and used as received. Synthesis of graphene supporting TiO 2 with reactive {001} facets (TiO 2 -G) [25] , [26] The graphene oxide (GO) was synthesized via a modified hummer’s method (Supplementary Methods) [54] . The lamellar protonated titanate (LPT) was used as the precursor of TiO 2 (Supplementary Methods). 2.5 g of wet LPT precursor and 30 mg GO (6 mg/mL) were dissolved in 15 mL of isopropyl alcohol by sonication for 30 min. Then, 0.5 mL of fluoric acid (40 wt%) and 16 mg of glucose were dropped into the solution under continuous stirring. The mixed solution was subjected to solvothermal treatment at 180 °C for 12 h. When the reaction system was cooled to room temperature, the black precipitate, TiO 2 -G, was washed thoroughly with water and ethanol, and then dispersed in absolute ethanol for the next step. Creation of porous composite structure by in situ knitting hypercrosslinked polymers on TiO 2 -functionalized graphene (HCP-TiO 2 -FG) Firstly, the phenyl-substituted graphene supporting TiO 2 (TiO 2 -FG) was obtained by the functionalization of graphene skeleton [55] . 5 millimoles of aniline (2 equivalent per graphene carbon), 100 mg TiO 2 -G, and 30 mL acetonitrile were added to a 50 mL round-bottom flask and stirred for 60 min. 5 millimoles of isoamyl nitrite was added under nitrogen atmosphere, and then the reaction mixture was heated with stirring to 80 °C for 24 h. The TiO 2 -FG was obtained by filtration and washing thrice with chloroform, further purified by extracting with chloroform for 24 h, and finally dried in a vacuum oven at 60 °C for 24 h. Secondly, the knitting process was performed as follows: under a N 2 atmosphere, the catalyst (AlCl 3 , 104 mg, 12 equiv syn -PhPh 3 ) was added to a mixture of syn -PhPh 3 (20 mg) and TiO 2 -FG (40 mg) in dichloromethane (8 mL), and then the system connected to nitrogen-line to form relatively less air-controlled environment. The reaction system was then stirred at 0 °C for 4 h, 30 °C for 8 h, 40 °C for 12 h, 60 °C for 12 h, and 80 °C for 24 h to obtain the resulting material. The resulting precipitate was quenched using HCl-H 2 O ( V /V = 2:1), and washed thrice with water and twice with ethanol, extracted with ethanol for 48 h, and finally dried in a vacuum oven at 65 °C for 24 h. The amount of syn -PhPh 3 was changed to 25 and 30 mg to adjust the thickness of HCP outer layers in the HCP-TiO 2 -FG composite structure. The resulting samples were labeled as HCP-TiO 2 -FG-1 and HCP-TiO 2 -FG-2, respectively. Synthesis of TiO 2 /HCP-FG composite For comparison, another type of composite, TiO 2 /HCP-FG, was prepared by a common synthetic method to illustrate the superiority of such well-defined HCP-TiO 2 -FG composite structure for CO 2 uptake. That is, syn -PhPh 3 was knitted on FG and then the HCP-FG was used as a supporting material for TiO 2 crystals growth. Firstly, hydrazine hydrate was used to reduce GO to graphene. GO (225 mg) was dispersed in 1 wt% aqueous sodium dodecylbenzene-sulfonate surfactant solution (225 mL) and sonicated for 60 min. The GO dispersion was reduced with 98% hydrazine hydrate (4.5 mmol) at 100 °C for 24 h after its pH was adjusted to 10 by 5% NaOH solution. Secondly, the HCP-FG was synthesized by the above diazonium salt process and solvent knitting method (20 mg FG and 20 mg syn -PhPh 3 ). Finally, the TiO 2 /HCP-FG composite was obtained by the same solvothermal process as TiO 2 -G by adding HCP-FG instead of GO. Photocatalytic test for CO 2 conversion Photocatalytic activity for CO 2 conversion of the synthesized catalysts was evaluated in a closed gas reactor. A 300 W Xe lamp was used as the light source. For visible light photocatalysis, a cutoff filter was used to remove any radiation below 420 nm. Before the photocatalytic reaction, the catalyst powder (20 mg) was placed in a circular glass dish that was positioned 8 cm away from the light source. The optical density was measured to be 433 mW cm −2 and the illuminated area of photocatalyst was about 3.14 cm 2 . The CO 2 was generated by the reaction of sodium hydrogen carbonate with diluted sulphuric acid after removing the air. The gas evolutions were analysed by gas chromatography (GC-2014CA, Shimadzu Corp., Japan). Characterization of materials FT-IR spectra were recorded on a Bruker Vertex 70 Spectrometer employing the KBr disk method. Thermogravimetric analysis (TGA) was performed from room temperature to 850 °C under nitrogen and air, employing a Perkin Elmer Instrument Pyris1 TGA with a heating rate of 10 °C min −1 . The field-emission scanning electron microscopy (FE-SEM) images were recorded employing a FEI Sirion 200 field-emission scanning electron microscope operated at 10 kV. The X-ray powder diffraction (XRD) (PANalytical B.V.) spectra were recorded by using an x’pert3 powder equipped with Cu Kα radiation at a scanning rate of 4° min −1 . X-ray photoelectron spectroscopy (XPS) measurements were performed on AXIS-ULTRA DLD-600W with an Al Ka source. The high-resolution transmission electron microscopy (HR-TEM) and scanning transmission electron microscopy (STEM) images of samples were recorded on a Tecnai G2 F30 microscope (FEI Corp. Holland). The High-Angle Annular Dark Field (HAADF) mapping images and three-dimensional TEM (3D-TEM) movie were obtained on a Talos F200X field-emission transmission electron microscope. The 3D-TEM movie in the Supplementary Movie 1 was created by taking multiple views of the sample at differ angles from −50° to 50° with 2° increments. The actual loading amount of Ti was measured by inductively coupled plasma-mass spectrometry (NexION 300X, Perkin Elmer). UV-vis diffuse reflectance spectra (DRS) were obtained on a scanning UV-vis spectrometer (LabRAM HR800) with integrating sphere detector. Gas (H 2 , N 2 , CO 2 ) sorption properties and specific surface area of samples were measured using a Micromeritics ASAP 2020 surface area and porosity analyzer. Before analysis, the samples were degassed at 110 °C for 8 h under vacuum of 10 −5 bar. Pore size distribution was calculated by N 2 adsorption isotherm employing the Tarazona nonlocal density functional theory (NLDFT) model assuming slit pore geometry. Total pore volumes ( V toal ) were derived from nitrogen sorption isotherms at relative pressure P/P 0 = 0.995. The mix gas adsorption experiment were checked by volumetric adsorption-gas chromatograph instrument BELSORP-VC. The samples were degassed at 100 °C for 8 h to remove the remnant solvent molecules before measurement. The pure water vapor adsorption experiment was investigated by moisture sorption analyser Hiden IGAsorp. The isotopic labelling was confirmed using a gas chromatography-mass spectrometry (SHIMADZU GCMS-QP2020). The Ultraviolet photoelectron spectroscopy (UPS) measurement was performed on a VG Scienta R4000 analyzer using a monochromatic He I light source (21.2 eV). A sample bias of −5 V was applied to observe the secondary electron cutoff (SEC).